Switching and amplification in disordered lasing resonators Controlling the flow of energy in a random medium is a research frontier with a wide range of applications. As recently demonstrated, the effect of disorder on the transmission of optical beams may be partially compensated by wavefront shaping, but losing control over individual light paths. Here we demonstrate a novel physical effect whereby energy is spatially and spectrally transferred inside a disordered active medium by the coupling between individual lasing modes. We show that it is possible to transmit an optical resonance to a remote point by employing specific control over optical excitations, obtaining a random lasing system, which acts both as a switch and as an amplifier. Nowadays, information is processed either electronically [1] or optically [2] , [3] , by using devices like transistors and optical modulators, which are also developing in many unconventional fashions [4] , [5] , [6] , [7] , [8] , [9] , [10] . However, the mechanisms underlying signal processing and transport in the presence of disorder are in many respects unknown even if they occur in numerous fields, such as biology, quantum networks, granular systems and many others [11] , [12] , [13] , [14] , [15] . There are several open questions regarding information transmission in complex systems, for example, which are the relevant degrees of freedom, which is the value of their mutual coupling and which is the way to route and control energy flow in presence of randomness. In linear optics, phase manipulation allows a monochromatic wavefront to be transmitted and focused beyond strongly scattering media [16] , [17] , [18] , but the actual light path cannot be affected. In the field of photonics, random lasers (RLs), that is, lasers based on disordered materials [19] , [20] , [21] , [22] , are highly non-linear, their modes exhibit variable spatial extent [23] and pronounced mutual interactions; thus, they are a fertile ground where long-range transport can be studied. In such open systems, the various forms of localization [24] are naturally coupled; thus, it must be possible transferring energy from one mode to another. Here we identify coupled resonances located at distant locations in an RL, measure their effective coupling in an absolute way and demonstrate switching, routing and amplification of a signal from one mode to another. Moreover, the results are theoretically interpreted in the framework of the coupled mode theory. The observed effect can be described in terms of an analogy between a field-effect transistor and an RL with two pump wedges working as controls, showing that signal amplification and all-optical gating can be achieved. Polychromatic interaction and amplification The first step to control modes interaction is to select individual modes with a controlled distance. We are able to control the set of modes pushed above threshold, and to influence their degree of localization by shaping the pump beam (see refs 23 , 25 , 26 and Methods section). We define three spatially separate regions of our cluster (named C1): the upper part is the source (S) area, the middle-lower part is the gate (G) area and the lower part is the drain area. Source and gate ( Fig. 1b ) may be activated (ON state) by pumping the corresponding wedge-shaped area, either individually ( Fig. 1a for S and Fig. 1b ) for G, or simultaneously ( Fig. 1c ), whereas drain is used only as a probe, to collect light (with a fibre). Thus, the cluster may be prepared in three different configurations: (1) S:ON; G:OFF, (2) S:OFF; G:ON and (3) S:ON; G:ON. In addition, light may be collected at the source (upper green spot in Fig. 1c ) or at the drain (lower blue spot in Fig. 1c ). 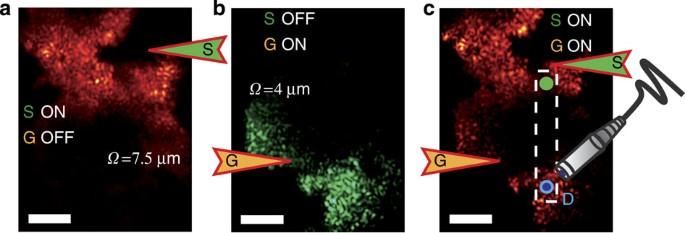Figure 1: All-optical disordered-based gate. Optical image of the intensity emitted by the titanium dioxide cluster in various pumping configurations: (a) source-only pumping, source mode is on, (b) gate-only pumping, drain mode is on, and (c) source and gate simultaneously. Scale bar, 5 μm. Figure 1: All-optical disordered-based gate. Optical image of the intensity emitted by the titanium dioxide cluster in various pumping configurations: ( a ) source-only pumping, source mode is on, ( b ) gate-only pumping, drain mode is on, and ( c ) source and gate simultaneously. Scale bar, 5 μm. Full size image The D and S signal from the cluster C1 pumped in three configurations are reported in Fig. 2 . Configuration S:ON; G:OFF ( Figs 1a and 2a ) reports completely different signals for S and D (in particular, no signal is observed at D). 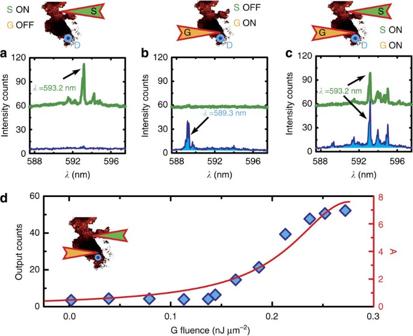Figure 2: Polychromatic action and amplification. Spectra measured at S (green line) and at D (azure line) in different pumping configurations: (a) S:ON; G:OFF; (b) S:OFF; G:ON; (c) S:ON; G:ON. Schemes atop each panel show the adopted configurations. (d) The intensity of the the S mode (λ=593.2 nm) measured at D as a function of pump fluence at the gate. The right y axis report amplification of the source signal measured as a function of the gate fluence, whereas the red solid line is the best fit to a Lorentzian accounting for the mode coupling. Figure 2: Polychromatic action and amplification. Spectra measured at S (green line) and at D (azure line) in different pumping configurations: ( a ) S:ON; G:OFF; ( b ) S:OFF; G:ON; ( c ) S:ON; G:ON. Schemes atop each panel show the adopted configurations. ( d ) The intensity of the the S mode ( λ =593.2 nm) measured at D as a function of pump fluence at the gate. The right y axis report amplification of the source signal measured as a function of the gate fluence, whereas the red solid line is the best fit to a Lorentzian accounting for the mode coupling. Full size image The opposite happens in Fig. 1b for configuration S:OFF; G:ON, and we find signal at the drain D but no signal at the source S. Furthermore, the signal at the drain has a spectral content, which bears no resemblance whatsoever with either spectrum in the previous configuration ( Fig. 2b ). Finally in Fig. 1c , the S and G wedges are both pumped (S:ON; G:ON), and we observe that the signal at the drain D has the same spectral content as that at the source S ( Fig. 2c ) and no resemblance with its former lineshapes in Fig. 2a or b , providing evidence that light in S has been routed to the drain region, with G acting as a gate. Recapitulating, we see that in the S:ON; G:OFF case, the S mode is clearly visible (showing a principal resonance at λ =593.2 nm), with no emission at the D position while in the S:OFF; G:ON case a resonance at λ =589.3 nm is found at the D position, with no emission from S. Hence, we find two modes located at different positions and with different spectra (with mode S being more spatially extended than mode D, localization length is reported in Fig. 1 ). When both modes are activated at the same time (S:ON; G:ON) a striking effect is provoked; although S is oscillating at its own frequency (thus independent of the state of G), the D mode is forced to oscillate at the very same frequency of S ( λ =593.2 nm). The resonance lying at S retains its frequency, but that at D can be driven by G to adopt the S spectral content. In other words, the spectral content of S is transported to D, when G is turned on. The amplification as a function of the control signal is reported in Fig. 2d right axis. We also stress that the process is inherently parallel and we notice that several wavelengths are simultaneously routed from to , as shown in the spectra in Fig. 2c . The switching process To understand the physical mechanisms underlying this controlled transport, we measured the spectrum at D as a function of the energy provided through the S wedge (when G is kept ON). 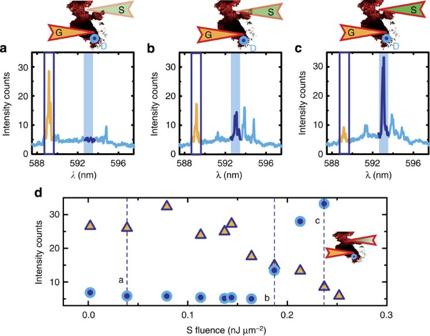Figure 3: The switching process. Spectrum obtained from the drain as a function of the energy at the source. The fluence at the source wedge is 0.04 nJ μm−2ina; 0.18 nJ μm−2inband 0.23 nJ μm−2inc. Paneldshows the intensity measured at D for the drain frequency (589.3 nm, triangles) and for the source frequency (593.2 nm, circles) as a function of the fluence at S. Data corresponding to the top panels are indicated. Figure 3a shows the retrieved average spectra (averaging over 25 single shots), revealing that the mode at D (excitable with the gate G:ON at λ =589.3 nm, blue rectangle) is steadily suppressed as the S mode (at λ =593.2 nm, azure-shaded area) gains intensity. Figure 3d displays the average G (S) mode intensity as full triangles (open circles), as a function of the fluence supplied through the S wedge. Vertical lines labelled a, b and c correspond to spectra in Fig. 3a . The progressive transfer of intensity from one mode to the other shows that above a certain threshold, energy is routed from the G to the S mode due to the onset of the the non-linear interaction and the competition between the involved modes. Figure 3: The switching process. Spectrum obtained from the drain as a function of the energy at the source. The fluence at the source wedge is 0.04 nJ μm −2 in a ; 0.18 nJ μm −2 in b and 0.23 nJ μm −2 in c . Panel d shows the intensity measured at D for the drain frequency (589.3 nm, triangles) and for the source frequency (593.2 nm, circles) as a function of the fluence at S. Data corresponding to the top panels are indicated. Full size image Further evidence of the switching process is reporter in the hyperspectral maps reported in Fig. 4 . Each map corresponds to a different pumping condition (see Methods), which allows to estimate the modes extension in the S:ON; G:OFF configuration in Fig. 4a , in the S:OFF; G:ON configuration in Fig. 4b and in the S:ON; G:ON configuration in Fig. 4c . Note that in the S:ON; G:ON configuration the intensity at the source frequency flows into the area corresponding to the drain, whereas the ‘gate-only’ peak disappears everywhere. 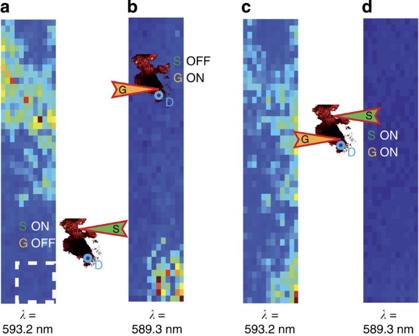Figure 4: Hyperspectral maps. Each map is obtained by fixing the indicated detection wavelength. Panelais relative to the configuration S:ON; G:OFF and shows the spatial extent of the source mode. Panelbshows S:OFF; G:ON, that is, the D mode that lies in and around where drain spectra are measured. Panelscanddare relative to the S:ON; G:ON configuration for the S and for the D modes, respectively. Figure 4: Hyperspectral maps. Each map is obtained by fixing the indicated detection wavelength. Panel a is relative to the configuration S:ON; G:OFF and shows the spatial extent of the source mode. Panel b shows S:OFF; G:ON, that is, the D mode that lies in and around where drain spectra are measured. Panels c and d are relative to the S:ON; G:ON configuration for the S and for the D modes, respectively. Full size image The random character of the system at hand makes its functioning unpredictable, meaning that each cluster presents its own set of modes with specific interactions so that finding modes that act as source, gate and drain requires inspection each time. Yet, the spatio-spectral transfer described has been found to occur in all clusters investigated. The adoption of the roles as source or drain, although requiring more research, seems to be essentially governed by the model size, the larger mode acting as source and dominating the spectral features of the drain. In very small clusters, the limited number of modes can be so small to preclude the observation of the switching. Coupled mode theory The phenomenon may be explained exploiting the coupled mode theory equations [27] for two individual interacting modes: a larger one (mode S, that is, the source mode) and a smaller one (mode D, that is, the drain mode). At small pumping for the drain mode, the equation for its complex amplitude reads: where , , , and are, respectively, the amplitude of the mode D, its resonance frequency, its gain and losses, and its degree of coupling with the source mode (whose intensity is referred as a ). When mode S is not pumped, the coupling term is negligible and mode D oscillates at its fundamental frequency. On the other hand, if energy in the larger mode is enough, one may search for a solution oscillating at the frequency of the S mode. In this case, after simple algebra (see Methods section) one finds that Equation shows that amplification follows a Lorentian lineshape when increasing the gain for the drain g (see Fig. 2d ) and reach a maximum value . Knowing maximum amplification and the frequency difference , one can use equation (2) to estimate the K constant. At saturation and defining , one obtains from equation (2): where is the modes difference in wavelength and K is the coupling measured in the units of wavelenght. In the case reported in Fig. 2 , the maximum amplification has a value of , and is 4.4 nm, resulting in a coupling constant of 11 nm, and the same number has been obtained from the fit with equation (2) (see Methods). is thus the spectral distance for two modes that allows for a maximum amplification of 1; spectrally closer modes may achieve higher amplifications, whereas more distant ones will be not amplified exactly like in the case of a mode forced to oscillate far from its resonance. This result is consistent with the fact that we observe an effective coupling between modes with a separation of the order of =5 nm. The range of the interaction The range over which spatial transfer from S to D is possible can be estimated by measuring how closely a drain spectrum with source ON resembles its natural state (source OFF) as a function of distance. 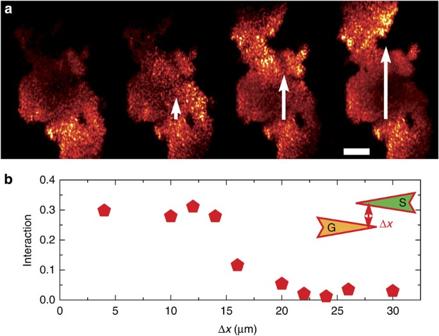Figure 5: Range of the interaction. (a) Images of the emission from the cluster C1 for different values of Δx, from left to right Δx=4, 12, 20, 30 μm; (b) interaction obtained from the spectral overlaps (see text) as a function of Δx. Scale bar, 5 μm. Figure 5 shows the degree of interaction (defined in the Methods section) as a function of gate to source distance Δ x for cluster C1. The interaction strength drops to 0 at distances larger than 15 μm. The top panels in Fig. 5 show the intensity distribution retrieved with various Δ x for small Δ x resonances (hotspots in the images) of D and S dwell in the same region, thus energy may flow freely between different modes. When Δ x is larger, a region with low pumping (and thus large losses) separates the two sets of hotspots impeding the transport. Figure 5: Range of the interaction. ( a ) Images of the emission from the cluster C1 for different values of Δ x , from left to right Δ x= 4, 12, 20, 30 μm; ( b ) interaction obtained from the spectral overlaps (see text) as a function of Δ x . Scale bar, 5 μm. Full size image In summary, by exploiting a selective excitation we have been able to put two lasing modes in the condition to feel a controllable cross-talk. A source and a drain mode have been put in connection by means of third mediator signal called gate, resulting in either a frequency switching and amplification at the drain. The results are quantitatively reproduced by a model based on coupled mode theory that allow to predict the energy behaviour and to measure the absolute way the coupling constant between disordered resonators. We have found that lasing modes in an RL can be made to interact, so that spectral features can be actively controlled and transported to remote locations by a control optical signal. Above a world of possible future applications for controlling light flow, the formulation of a consistent model for the interaction of modes, and the first measurement of the inter-mode coupling constant, is a milestone, which will allow to unravel its underlying physics and the nature of switching between different RL regimes. Moreover, the investigation of the interaction between two disordered lasing resonances, allows to put the basis for a comprehensive description of the random lasing phenomenon, also at the macroscopic level in which the amount of modes is huge and their couplings countless. Future challenges will be the study of the switching close to the Anderson regime, where the energy flow between two resonances is inhibited and the investigation of the nature of the interaction between localized and delocalized states. Samples and experimental setup The system considered is a cluster of titanium dioxide nanoparticles embedded in a rhodamine solution, which acts as the optically amplifying medium under excitation by a laser-pump beam at wavelength =532 nm. This disordered device comprises many nanoparticles that self-assemble to form the multi-mode optical resonator. By tailoring the spatial profile of the pump beam, we control the activated modes; the directional pumping determines the spatial regions of the cluster, which are pushed above threshold, and their degree of localization, that is, the spatial extension of the involved electromagnetic resonances [23] , [25] , [26] . This is achieved by exploiting a scheme in which the shape of the pumped region generates stimulated emission engineered to hit the cluster at pre-defined points in pre-defined directions. The pumped area comprises two wedges of fixed orientation and controllable relative position and angular aperture (triangular arrows in Fig. 1 ) and a superimposed circular spot (not shown). The two wedges are parallel, pointing in opposite directions, and vertically shifted by an amount Δ x (Δ x =15 μm in Fig. 1 ). In this way we are able to activate modes at a desired location and, for each mode, we control the localization length by the angular spread of the wedges [23] . A motor-controlled translator has been used to obtain hyperspectral maps in Fig. 4 . The measurement is performed by moving the fibre in the image plane with nanometre resolution, thus obtaining the spectra emitted at every point of the map by a circular region of the cluster (one disk of 1 μm in diameter). The maps contain more information than the simple measurement at the drain and source edges of the cluster, depicting how the modes are organized after the activation of a close neighbour.We studied, in particular, an area represented by the dotted rectangle in Fig. 1 . The rectangle configuration in particular has been chosen, because it allows to cover the area that includes the two modes (source on one edge of the rectangle and drain at the other). Measuring amplification In our disordered photonic device, we are able to transfer spectral features from the source to the drain edge of the cluster by activating the gate. An important parameter that needs careful measurement is the rate of signal amplification, that is, the amount of intensity transferred through the drain mode (obtained for S:ON; G:ON at the source frequency λ =593.2 nm for sample C1) as compared with the signal at the same frequency at the D edge of the cluster when just the S is on (S:ON; G:OFF). Even when the G is OFF, the source alone is able to transfer a small signal to the drain. The signal is so small that particular features cannot be noticed in the total spectrum ( Fig. 2 ). An estimate is given by the average intensity in the hyperspectral map ( Fig. 4a ; that is, for λ =593.2 nm) in the area corresponding to the drain mode (individuated by the dashed square). The value of the amplification depends from value of the intensity of the S mode in different configurations Coupled modes theory interpretation and data fitting The switching process results from the coupling between modes. Following the approach of Haus [27] and neglecting high-energy non-linear saturation effects, the differential equations driving the amplitude of two modes, one larger (mode S) and one smaller (mode D), read as where , , , and are, respectively, the amplitude of the mode D, its resonance frequency, its gain and losses, whereas the symbols bearing S label represent the same physical quantities for the source mode. If D is much smaller in extension than the mode S, the coupling term in the first equation ( ) may be neglected. On the other hand, this is never true for the D mode. In the extreme case in which the coupling term is much stronger than the part oscillating at the master frequency, one may search solutions oscillating at . Substituting the solution in equation 4, one finds from which The amplification defined as results to be This Lorenzian describes the behaviour of A as a function of the the gain (related to external pumping) and of the frequency difference . At very small , amplification is negligible. When approaches , gain compensates losses and the amplification reaches a maximum that is infinite on resonance ( ) and lowers with increasing detuning. Equation (7) may be used to fit directly the data of Fig. 2 . In the fit, we left as a free parameter the coupling parameter and a scaling factor for the pumping (effective pumping of the mode is proportional to the laser energy density per pulse). By this approach, the retrieved value is about 11 nm, which is consistent with what was retrieved experimentally; interacting modes were always found between 2 and 5 nm. Interaction range A method to determine the range of the interaction is to quantify how much the spectrum emitted by the drain changes by switching on the source as a function of the distance Δ x between the source and the drain. If the activation of the source results in a lineshape modification of the spectrum at D, their interaction is proved. Conversely, if the source is at a distant position, such that its activation does not affect D, then the interaction is weak or absent. The actual measurement of the interaction is performed by collecting the spectrum at D in two configurations: configuration 1 is S:OFF; G:ON and configuration 2 is S:ON; G:ON. The spectra obtained from these two measurements have to be compared quantitatively to retrieve the degree of similitude. This is done by calculating the normalized overlap (normalized such that ). Two identical spectra will show a value of Q equal to 1, whereas two different spectra will approach 0. Thus, in a non-interacting case, turning S ON will produce no change in the spectrum and , whereas in a strong interacting case the addition of the S wedge will produce large changes in the D spectrum leading to lower values of Q . The minimum value of Q retrieved for the strongly interacting configuration is 0.7. This residual value is because of the fact that a large part of the emission is due to fluorescence, which is repeatable and independent on the particular shape of modes or from interaction; however, a clear change of the Q -value is clearly evidenced as a function of Δ x and nearly no residual interaction is measurable for values above 25 μm. A more user-friendly observation is the interaction obtained as 1− Q . This is plotted in Fig. 5 for the cluster C1. Occurrence of the switching phenomenon An important issue is the occurrence of the switching phenomenon. Here we give a quantitative estimation of how many switchable modes may be found in an individual cluster (we considered clusters with an average diameter between 15 and 35 μm). If isolation procedure has been performed [25] , all the isolated clusters possess modes that may be activated nearly from every input direction [26] and with a threshold between 0.01 and 0.5 nJ μm − . This means that for every value of , we are able to activate some modes of the cluster. Usually, close to the lasing threshold and for small values of the wedge angular span , a single mode may be activated per acceptance angle (0.5°). The first challenge is to find a mode of large size that will work as a source. This may be found by performing a scan in of the emitted spectrum and by controlling the area illuminated on the cluster. We found a mode with Ω >7 μm every 20 scanned values of . The average localization length being about Ω~ 3 μm, the selected source mode will be much larger than the majority of all other modes. Considering the average mode acceptance of RL modes one can find at least thirty modes able to act as source. Once a proper source is found, one has to find a mode that is able to act as a drain; this is done by placing the gate wedge at about Δ x =15 μ m (the average interaction length, see Fig. 5 ) from S and scanning in . For each value of , one has to try with both S:OFF; G:ON and with S:ON; G:ON configuration, searching for a drain mode switching at the source frequency. The accessible configurations that may be tested are of the order of 360 to which one has to add various values of Δ x and of that may be also scanned. Thus, in all the isolated clusters, the probability to not find any mode coupled with a certain source is negligible. How to cite this article: Leonetti M. et al . Switching and amplification in disordered lasing resonators. Nat. Commun. 4:1740 doi: 10.1038/ncomms2777 (2013).